KRAS allelic imbalance drives tumour initiation yet suppresses metastasis in colorectal cancer in vivo 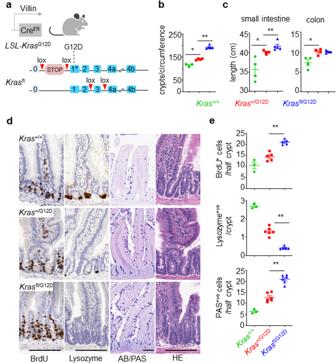Fig. 1: Wild-typeKrasdeletion altersKrasG12Dmutant intestinal homoeostasis. aSchematic representing the generation ofKrasfl/G12Dmice: Villin Cre, Cre recombinase; ER oestrogen receptor; lox, Cre-Lox recombination site; LSL Lox-Stop-Lox cassette. Created with BioRender.com.bNumber of crypts per circumference from at least 25 of the small intestine ofKras+/+,Kras+/G12DandKrasfl/G12Dmice, sampled 30 days post Cre-induction (Kras+/+,n= 3, 2M,1F;Kras+/G12D,n= 4, 2M, 2F; andKrasfl/G12D,n= 5, 4M, 1F). Data are ± s.e.m. *P= 0.0286, **P= 0.0079, one-way Mann–WhitneyUtest. Experiments carried out on C57BL/6J background ≥ N2.cLength (cm) of small intestine (SI) and colon ofKras+/+,Kras+/G12DandKrasfl/G12Dmice, sampled 30 days post Cre-induction (Kras+/+,n= 4, 3M, 1F;Kras+/G12D,n= 4, 2M, 2F; andKrasfl/G12D,n= 5, 3M, 2F). Data are mean ± s.e.m. *P= 0.0143, **P= 0.0079 one-way Mann–WhitneyUtest. Experiments carried out on C57BL/6J background ≥ N2.dRepresentative 5-bromo-2′-deoxyuridine (BrdU), Lysozyme, Alcian blue/periodic acid-Schiff (AB/PAS) and H&E staining ofKras+/+,Kras+/G12DandKrasfl/G12Dmouse small intestine, sampled 30 days post Cre-induction. Scale, 100 μm.eTop: Number of BrdU-positive cells from at least 25 half-crypts in SI from (d). Data are mean ± s.e.m, (Kras+/+,n= 3, 2M, 1F;Kras+/G12D,n= 5, 3M, 2F;Krasfl/G12Dn= 5, 3M, 2F), **P= 0.004, one-way Mann–Whitney U test. Middle: Number of Lysozyme-positive cells from at least 25 crypts in SI ofKras+/+,Kras+/G12DandKrasfl/G12Din SI from (d) Data are mean ± s.e.m, (Kras+/+,n= 3, 2M, 1F;Kras+/G12D,n= 6, 3M, 3F;Krasfl/G12Dn= 5, 3M, 2F), **P= 0.0022, one-way Mann–Whitney U test. Bottom: Number of PAS-positive cells from at least 25 half-crypts in SI.Kras+/+,Kras+/G12DandKrasfl/G12Din SI from (d) Data are mean ± s.e.m, (Kras+/+,n= 3, 2M, 1F;Kras+/G12D,n= 6, 4M, 2F;Krasfl/G12Dn= 6, 4M, 2F). **P= 0.0011, one-way Mann–WhitneyUtest. Experiments carried out on C57BL/6J background ≥ N2. Source data are provided as a Source Data file. Oncogenic KRAS mutations are well-described functionally and are known to drive tumorigenesis. Recent reports describe a significant prevalence of KRAS allelic imbalances or gene dosage changes in human cancers, including loss of the wild-type allele in KRAS mutant cancers. However, the role of wild-type KRAS in tumorigenesis and therapeutic response remains elusive. We report an in vivo murine model of colorectal cancer featuring deletion of wild-type Kras in the context of oncogenic Kras . Deletion of wild-type Kras exacerbates oncogenic KRAS signalling through MAPK and thus drives tumour initiation. Absence of wild-type Kras potentiates the oncogenic effect of KRASG12D, while incidentally inducing sensitivity to inhibition of MEK1/2. Importantly, loss of the wild-type allele in aggressive models of KRASG12D-driven CRC significantly alters tumour progression, and suppresses metastasis through modulation of the immune microenvironment. This study highlights the critical role for wild-type Kras upon tumour initiation, progression and therapeutic response in Kras mutant CRC. It is known that oncogene allelic imbalance is a frequent event in cancer cells, known to impact key oncogene loci such as KRAS and BRAF [1] . These allelic imbalances can result from genomic gains or losses, focal amplifications at the oncogene loci or loss of heterozygosity impacting the wild-type allele. Nonetheless, the functional and therapeutic consequences of such imbalances are poorly understood. Mutations in KRAS oncogene are frequently detected in many cancers, including colorectal adenocarcinoma (CRC) and pancreatic ductal adenocarcinoma (PDAC). Hotspot mutations involving codons 12, 13, 61 and 146 of KRAS lead to constitutive activation of KRAS and hyperactivation of many downstream effector signalling pathways, including MAPK and PI3K-AKT pathways [2] , [3] . Biochemically, these hotspot mutations have been shown to increase the abundance of GTP-bound active KRAS, through altered GTP hydrolysis and nucleotide exchange rates based on the type of mutation [4] . Recent reports have shown that as a likely consequence of their distinct biochemical properties, each specific KRAS mutation has a unique transforming potential and tumour-promoting capacity dependent on the tissue or cancer type [5] , [6] , [7] . It is now well established that the frequency of KRAS mutation differs widely based on the tissue of origin (40% of CRC and 93% of pancreatic cancers) [8] . We and others have previously shown that oncogenic Kras cooperates with Apc loss in driving colorectal tumorigenesis [9] , [10] , [11] . The majority of studies to date have focused on gain-of-function effects of KRAS mutations [12] . Unfortunately, and despite the recent successes with KRASG12C isoform-specific inhibitors, it is widely accepted that mutant KRAS is strongly associated with resistance to therapies, particularly those targeting upstream or downstream signalling nodes such as EGFR, MEK, PI3K and mTOR [13] , [14] , [15] . This said, given their position at the nexus of many key oncogenic and growth-promoting signalling pathways, significant efforts are underway both to directly target mutant RAS oncoproteins, and to target signalling through the wild-type molecule [16] , [17] . Recent work from several labs has highlighted the heterogeneous properties of KRAS alterations in human cancer, having successfully modelled a spectrum of KRAS mutations in relevant model systems [5] , [6] , [7] . In addition to this spectrum of oncogenic KRAS mutations, evaluation of specific pro- or anti-tumourigenic roles for the wild-type RAS proteins in the context of oncogenic RAS across cancer types has been controversial. It has previously been proposed that wild-type KRAS can exhibit tumour-suppressive characteristics in cancer [18] . More recently, it was also shown that KRAS dimerization is required for the function of oncogenic KRAS [19] . In addition, it has become clear that copy number alterations at KRAS such as copy number gain at the mutant allele, loss of heterozygosity, or broader allelic imbalance can result in enhanced fitness of cancer cell lines [1] , [20] , [21] , [22] . Indeed, it has been demonstrated that KRAS gene dosage can determine phenotypic characteristics and influence outcome of pancreatic cancer models in vivo [23] , [24] . Nonetheless, a clear understanding of the mechanistic basis of wild-type KRAS function in the processes of tumour initiation and progression of KRAS mutant tumours is yet to be defined. Understanding the function of wild-type KRAS is essential to identify effective therapeutic strategies for oncogenic KRAS -driven cancers and potential mechanisms of resistance to KRAS targeting therapies. Here, we demonstrate a critical role for wild-type KRAS in tumour initiation and progression of mutant KRAS-driven tumours. Using genetically engineered mouse models (GEMMs), we show that in the presence of an oncogenic Kras allele loss of the wild-type Kras allele augments oncogenic Kras signalling, leading to increased tumour initiation in vivo. Furthermore, utilising KRAS-driven colorectal cancer models we show that loss of wild-type KRAS promotes sensitivity to MEK inhibition in vivo. Finally, we show that deletion of wild-type Kras allele significantly alters the progression of advanced late-stage KRAS-driven colorectal tumours. Collectively, our studies provide important insights into KRAS biology and reveal a critical role for wild-type KRAS in the therapeutic resistance of KRAS-driven cancers. Allelic balance of mutant and wild-type KRAS affects homoeostasis in the murine intestine To accurately model the contribution of wild-type KRAS in CRC, we designed a GEMM that allows selective deletion of the wild-type Kras while expressing an oncogenic Kras LSL-G12D allele (hereafter Kras G12D ). Here, the wild-type Kras allele is replaced by a conditional Kras flox allele to generate Kras fl/LSL-G12D (hereafter referred to as Kras fl/G12D ) (Fig. 1a ). Recombination of these alleles is targeted to the intestinal epithelium through activity of a tamoxifen-inducible Cre recombinase, expressed under the control of the Villin promoter (villin-creERT2) (Fig. 1a ). Using this model we confirmed the impact of the oncogenic Kras G12D mutation upon intestinal epithelial homoeostasis, and subsequently went on to characterise any modification of this phenotype elicited by Kras fl/G12D . Intestinal tissue was sampled from mice at 30 days post-induction, with mutant KRAS found to promote enterocyte proliferation and robustly suppress Paneth cell differentiation in the small intestine as a consequence of increased MAPK signalling, consistent with previous reports [25] (Fig. 1b–e ). These features are further exacerbated by deletion of the wild-type copy in Kras fl/G12D mice, exemplified by increased proliferation in the intestinal crypt (BrdU + ) (Fig. 1d, e ). Moreover, Lysozyme and periodic acid-Schiff (PAS) or Alcian blue (AB) stains indicated further suppression of the Paneth cell lineage and increased abundance of secretory goblet cells (Fig. 1d, e ). These in vivo data are suggestive of a role for wild-type KRAS in restraining the impact of oncogenic KRAS mutation on the intestinal epithelium, which in turn translates into quantitative phenotypic differences. Fig. 1: Wild-type Kras deletion alters Kras G12D mutant intestinal homoeostasis. a Schematic representing the generation of Kras fl/G12D mice: Villin Cre, Cre recombinase; ER oestrogen receptor; lox, Cre-Lox recombination site; LSL Lox-Stop-Lox cassette. Created with BioRender.com. b Number of crypts per circumference from at least 25 of the small intestine of Kras +/+ , Kras +/G12D and Kras fl/G12D mice, sampled 30 days post Cre-induction ( Kras +/+ , n = 3, 2M,1F; Kras +/G12D , n = 4, 2M, 2F; and Kras fl/G12D , n = 5, 4M, 1F). Data are ± s.e.m. * P = 0.0286, ** P = 0.0079, one-way Mann–Whitney U test. Experiments carried out on C57BL/6J background ≥ N2. c Length (cm) of small intestine (SI) and colon of Kras +/+ , Kras +/G12D and Kras fl/G12D mice, sampled 30 days post Cre-induction ( Kras +/+ , n = 4, 3M, 1F; Kras +/G12D , n = 4, 2M, 2F; and Kras fl/G12D , n = 5, 3M, 2F). Data are mean ± s.e.m. * P = 0.0143, ** P = 0.0079 one-way Mann–Whitney U test. Experiments carried out on C57BL/6J background ≥ N2. d Representative 5-bromo-2′-deoxyuridine (BrdU), Lysozyme, Alcian blue/periodic acid-Schiff (AB/PAS) and H&E staining of Kras +/+ , Kras +/G12D and Kras fl/G12D mouse small intestine, sampled 30 days post Cre-induction. Scale, 100 μm. e Top: Number of BrdU-positive cells from at least 25 half-crypts in SI from ( d ). Data are mean ± s.e.m, ( Kras +/+ , n = 3, 2M, 1F; Kras +/G12D , n = 5, 3M, 2F; Kras fl/G12D n = 5, 3M, 2F), ** P = 0.004, one-way Mann–Whitney U test. Middle: Number of Lysozyme-positive cells from at least 25 crypts in SI of Kras +/+ , Kras +/G12D and Kras fl/G12D in SI from ( d ) Data are mean ± s.e.m, ( Kras +/+ , n = 3, 2M, 1F; Kras +/G12D , n = 6, 3M, 3F; Kras fl/G12D n = 5, 3M, 2F), ** P = 0.0022, one-way Mann–Whitney U test. Bottom: Number of PAS-positive cells from at least 25 half-crypts in SI. Kras +/+ , Kras +/G12D and Kras fl/G12D in SI from ( d ) Data are mean ± s.e.m, ( Kras +/+ , n = 3, 2M, 1F; Kras +/G12D , n = 6, 4M, 2F; Kras fl/G12D n = 6, 4M, 2F). ** P = 0.0011, one-way Mann–Whitney U test. Experiments carried out on C57BL/6J background ≥ N2. Source data are provided as a Source Data file. Full size image Allelic imbalance is reported to be a common feature associated with many oncogenes in addition to KRAS [1] . For example, BRAF allelic imbalance is reported to occur in 40% of BRAF mutant skin cancers [26] . Therefore, we tested whether Braf allelic imbalance could also impact intestinal homoeostasis. Here, we assessed the impact of a conditional oncogenic Braf V600E allele, alone or in combination with a conditional Braf targeting allele (henceforth referred to as Braf fl/V600E ), or when bred to homozygosity ( Braf V600E/V600E ), again under the control of villin-creERT2. To assess the impact of Braf V600E gene dosage, intestinal tissues were sampled from Braf +/V600E , Braf fl/V600E , Braf V600E/V600E or control mice at a time point 3 days post-induction recombination. As previously reported, we found that Braf V600E/+ promotes proliferation in the intestinal crypt (BrdU + ), indeed to a greater degree than Kras G12D/+ at this time point (Supplementary Fig. 1a, b ) [27] , [28] . In line with the phenotypes observed in KRAS mutant intestine, we find that altering allelic balance in favour of oncogenic Braf , either through breeding to homozygosity ( Braf V600E/V600E ), or through conditional deletion of the wild-type allele ( Braf fl/V600E ) leads to significant increase in crypt cell proliferation and loss of Lysozyme-positive Paneth cells (Supplementary Fig. 1a, b ). However, BRAF activation does not significantly alter the abundance of secretory goblet cells in the intestinal epithelium (Supplementary Fig. 1a, b ). Collectively, these data show that allelic imbalance at oncogene loci akin to that seen in human cancer exacerbates specific oncogene-associated and cancer-related phenotypes. Wild-type Kras deletion in the presence of oncogenic KRASG12D and Wnt activation accelerates tumorigenesis via MAPK signalling Given the observed impact upon normal intestinal homoeostasis driven by altered gene dosage at oncogenic loci, we investigated whether these events might cooperate with the concomitant loss of the tumour suppressor gene Apc . The Kras fl/G12D mouse line described above was bred to the well-characterised mouse line bearing conditional deletion of the tumour suppressor gene Apc (villin-creERT2 Apc fl/fl ), generating Apc fl/fl Kras fl/G12D or Apc fl/fl Kras +/G12D mouse lines as simple, tractable models of oncogene-induced hyperproliferation in vivo. Homozygous deletion of Apc in the murine intestine results in a robust phenotype, driven by hyperproliferation and altered differentiation of the intestinal crypt epithelium [29] . Moreover, we have shown that this phenotype is exacerbated by expression of oncogenic Kras [10] , [11] . Using this system, we investigated whether loss of wild-type Kras , in the context of an oncogenic Kras G12D mutation and Apc loss, impacted epithelial proliferation in vivo. Indeed, this was the case with significantly enhanced proliferation, as denoted by BrdU incorporation, observed in the intestinal epithelium of Apc fl/fl Kras fl/G12D mice when compared to Apc fl/fl Kras +/G12D mice (Fig. 2a, b ), with the area of proliferative cells extending higher in the villus epithelium in Apc fl/fl Kras fl/G12D mice. This was not due to Kras copy number or allele changes as confirmed using droplet PCR (Supplementary Fig. 2a, b ). The ectopic proliferation/dedifferentiation of cells in the villus epithelium is a key feature of Kras G12D mutation in the context of Apc deficiency, and is concomitant with an acquired ability of mutant cells to form organoid cultures in vitro [11] . Consistent with the observed proliferation in the villus epithelium of Apc fl/fl Kras fl/G12D mice, the characteristic organoid forming capacity was enhanced when compared to Apc fl/fl Kras +/G12D mice (Supplementary Fig. 2c, d ). These data indicate that loss of the wild-type copy of Kras in the context of concomitant oncogenic Kras G12D mutation and Apc depletion can enhance a number of Kras G12D associated phenotypes. Fig. 2: Wild-type Kras deletion increases proliferation, active KRAS and MAPK signalling. a Representative H&E and BrdU IHC of Apc fl/fl Kras +/G12D and Apc fl/fl Kras fl/G12D mice sampled 3 days post Cre-induction. Arrowheads indicate de-differentiating cells in the villi. Scale, 100 μm. b Boxplots showing BrdU-positive cells from at least 25 half-crypts in SI in Apc fl/fl , Apc fl/fl Kras +/G12D and Apc fl/fl Kras fl/G12D mice. Boxes depict interquartile range, central line indicates median and whiskers indicate minimum/maximum values (Apc fl/fl , n = 6, 4M, 2F ; Apc fl/fl Kras +/G12D , n = 6, 2M, 4F; and Apc fl/fl Kras fl/G12D , n = 5, 1M, 4F mice). ** P = 0.0022, ** P = 0.0043. c RAF-Ras Binding Domain (RBD) agarose affinity purification assay of three biologically independent samples per condition from Apc fl/fl Kras +/G12D and Apc fl/fl Kras fl/G12D intestinal organoids. Pulldown of RAS-GTP with RAF-RBD agarose beads. Top: Precipitates were immunoblotted using a pan-RAS antibody and input pan-RAS served as loading control. RAS-GTP activation levels were quantified and normalised to pan-Ras loading control. Apc fl/fl Kras +/G12D , n = 3, 2M, 1F; and Apc fl/fl Kras fl/G12D , n = 3, 1M, 2F. Bottom: Precipitates were immunoblotted using a KRASG12D antibody and input KRASG12D served as loading control. KRASG12D-RAF-RBD levels were quantified and normalised to KRASG12D loading control. Apc fl/fl Kras +/G12D , n = 3, 3M; and Apc fl/fl Kras fl/G12D , n = 3, 1M, 2F. d Quantification of RAF-RBD assay (left) and KRASG12D immunoblot (right from c ), ** P = 0.0045 (pan-RAS), ** P = 0.0044 (KRASG12D). e qRT-PCR analysis of Etv5, Etv4, Dusp4, Dusp5 and Spry3 in Apc fl/fl Kras +/G12D ( n = 6, 3M, 3F) and Apc fl/fl Kras fl/G12D ( n = 5, 1M, 4F) intestinal organoids. Data are mean ± s.e.m. Transcript levels were normalised to Gapdh . * P = 0.0260 ( Spry3 ) * P = 0.0411 ( Dusp5 ). f Left: Immunoblots showing PTEN, pAKT (Ser473), AKT, pERK1/2, ERK1/2, pMEK1/2, MEK1/2 and ß-actin in Apc fl/fl Kras +/G12D and Apc fl/fl Kras fl/G12D intestinal organoids. 6 Apc fl/fl Kras +/G12D and 5 Apc fl/fl Kras fl/G12D biological replicates per group, each lane represents organoids generated from individual mice from genotype indicated. Right: Quantification of immunoblots, phosphorylated proteins were normalised to total protein levels. Data are mean ± s.e.m. ** P = 0.0043 (pERK/ERK), * P = 0.0152 (pMEK/MEK), ** P = 0.0087 (pAKT/AKT), * P = 0.015 (PTEN/ß-actin). b , d , e , f using one-way Mann–Whitney U test. Source data are provided as a Source Data file. Full size image We hypothesised that loss of the wild-type Kras allele may alter baseline gene dosage of the oncogenic mutant allele, and as a result, lead to enhanced KRAS activation and increased signalling flux through downstream effector pathways and any associated feedback loops. This hypothesis was tested through comparison of organoid cultures derived from Apc fl/fl Kras fl/G12D and Apc fl/fl Kras +/G12D intestinal tissues. Initially, we quantified the relative proportion of GTP-bound, active RAS proteins. In these pull-down assays, Apc fl/fl Kras fl/G12D organoids were characterised by enhanced binding of RAS to the RAS-binding domain (RBD) of BRAF, when compared to Apc fl/fl Kras +/G12D , suggestive of a larger pool of active RAS (Fig. 2c, d ). It is well known that increased RAS activity translates into increased activation of downstream effector pathways such as the MAPK cascade [30] . To determine whether MAPK activity was increased in Apc fl/fl Kras fl/G12D and Apc fl/fl Kras +/G12D organoids, we quantified expression of known ERK-regulated transcripts, finding these to be enriched in Apc fl/fl Kras fl/G12D organoids (Fig. 2e ). To evaluate MAPK activity in more depth, we assessed downstream effector activity in these lines through quantitative immunoblotting. We detected a clear increase in phosphorylation of ERK1/2 and MEK1/2 in Apc fl/fl Kras fl/G12D organoids, with phosphorylation of AKT and expression of PTEN also elevated (Fig. 2f ). These data indicate that loss of the wild-type copy of Kras enhances the relative activity of the oncogenic mutant allele and drives downstream effector pathway signalling. Given the robust impact of wild-type Kras deletion in the acute setting above, we next addressed the role of wild-type KRAS on oncogenic KRASG12D-driven intestinal tumorigenesis. To this end, we generated villin-creERT2 Apc fl/+ Kras +/G12D (henceforth AKras +/G12D ) and villin-creERT2 Apc fl/+ Kras fl/G12D (henceforth AKras fl/G12D ). In this setting, intestinal tumour development occurs following sporadic loss of the second copy of Apc in individual intestinal crypts. Targeted mutation in the intestinal epithelium was induced through intraperitoneal administration of tamoxifen, with deletion of wild-type Kras in the context of oncogenic Kras G12D ( AKras fl/G12D ) resulting in a significant acceleration of tumorigenesis, and a consequent reduction of median survival based upon an endpoint defined by clinical signs associated with tumour burden. (Fig. 3a ). The reduced time to onset of signs associated with intestinal tumorigenesis in AKras fl/G12D mice was coincident with a striking tumour initiation phenotype, with development of numerous small lesions observed principally in the small intestine (Fig. 3b ). The initiating lesions observed in AKras fl/G12D mice were histopathologically comparable to those observed in AKras +/G12D mice (Fig. 3c ), and as expected, were positive for nuclear β-catenin (Fig. 3d ). Immunohistochemical analysis demonstrated nuclear accumulation of phosphorylated ERK1/2 (Fig. 3d ), increased expression of c-MYC and increased abundance of γH2AX in AKras fl/G12D tumours when compared to AKras +/G12D tumours, suggestive of MAPK pathway activation, increased cellular proliferation and activation of DNA damage response pathways (Fig. 3e, f ). Indeed, using BrdU incorporation as a marker for cellular proliferation, we demonstrated that the tumour epithelium of AKras fl/G12D mice is markedly more proliferative than that of AKras +/G12D mice (Fig. 3g ). Together, these results show that loss of the wild-type copy of Kras increases activity and signalling of the oncogenic mutant allele driving tumour initiation. Fig. 3: Loss of wild-type Kras increases mutant KRAS-driven tumourigenesis together with Apc loss. a Kaplan–Meier survival curve of villin-creERT2 Apc +/fl Kras +/G12D ( A Kras +/G12D ) and villin-creERT2 Apc +/fl Kras fl/G12D ( A Kras fl/G12D ) mice aged until clinical endpoint ( Apc +/fl Kras +/G12D , n = 8, 5M, 3F, MS, median survival = 63; Apc +/fl Kras fl/G12D , n = 9, 5M, 4F, MS, median survival = 25), **** P = 7.5 × 10 -5 , log-rank (Mantel-Cox) test. b Left: Boxplots showing total number of tumours from Apc +/fl Kras +/G12D and Apc +/fl Kras fl/G12D mice aged until clinical endpoint in SI and Colon. Right: Boxplots showing tumour area (mm 2 ) and tumour size (mm 2 ) in Apc +/fl Kras +/G12D and Apc +/fl Kras fl/G12D mice aged until clinical endpoint. Boxes depict interquartile range, central line indicates median and whiskers indicate minimum/maximum values ( Apc +/fl Kras +/G12D , n = 7, 5M, 2F; Apc +/fl Kras fl/G12D n = 5, 3M, 2F). ** P = 0.0013 (SI), ** P = 0.0013 (colon), * P = 0.036 (area), ** P = 0.0088 (size), one-way Mann–Whitney U test. c Representative H&E images of A Kras +/G12D ( n = 5, 2M, 3F) and A Kras fl/G12D ( n = 8, 5M, 3F) tumour. Dashed box highlights selected area shown in high magnification. d Representative images of nuclear β-catenin and pERK1/2 staining in Apc +/fl Kras +/G12D ( n = 5, 2M, 3F) and Apc +/fl Kras fl/G12D ( n = 8, 5M, 3F) tumours at clinical endpoint. Scale, 100 µm. e Representative images of γH2AX and c-MYC staining in Apc +/fl Kras +/G12D ( n = 5, 2M, 3F) and Apc +/fl Kras fl/G12D ( n = 8, 5M, 3F) tumours at clinical endpoint. Scale, 100 µm. f H-score of γH2AX ( Apc +/fl Kras +/G12D , n = 6, 4M, 2F; Apc +/fl Kras fl/G12D n = 5, 3M, 2F) and c-MYC ( Apc +/fl Kras +/G12D , n = 5, 2M, 3F; Apc +/fl Kras fl/G12D n = 8, 5M, 3F) IHC staining of ( e ). Boxes depict interquartile range, central line indicates median and whiskers indicate minimum/maximum values. ** P = 0.0043, *** P = 0.0008, one-way Mann–Whitney U test. g Representative BrdU staining of Apc +/fl Kras +/G12D and Apc +/fl Kras fl/G12D small intestinal tumours at clinical endpoint. Scale, 100 µm. Right: quantification of BrdU positivity in tumour cells. Boxes depict interquartile range, central line indicates median and whiskers indicate minimum/maximum values. ( Apc +/fl Kras +/G12D , n = 5, 3M, 2F; Apc +/fl Kras fl/G12D n = 4, 2M, 2F). * P = 0.0317, one-way Mann–Whitney U test. Source data are provided as a Source Data file. Full size image Loss of wild-type KRAS restores sensitivity to MEK inhibition in colorectal tumours in vivo We have demonstrated that altered allelic balance of oncogenic Kras G12D has a substantial impact upon tumour initiation in models of intestinal disease. Given that KRAS mutation is clinically associated with resistance to targeted therapies, we next investigated whether therapeutic efficacy is positively or negatively influenced by allelic imbalance at the Kras locus. We have previously shown that the observed intestinal crypt epithelium hyperproliferation characteristic of the Apc fl/fl Kras +/G12D model is resistant to MEK inhibition [11] , [31] , and that this proliferation is enhanced in Apc fl/fl Kras fl/G12D mice concomitant with increased KRAS and MAPK activity (Fig. 2c, f ). We reasoned that this increased MAPK activation might result in an acquired sensitivity to inhibition of MEK1/2 with a clinically relevant targeted therapeutic agent (AZD6244/selumetinib). As previously, we found that treatment of Apc fl/fl Kras +/G12D mice with AZD6244 had no impact upon intestinal hyperproliferation. Importantly, and in contrast, treatment with AZD6244 not only significantly decreased proliferation in the intestinal crypt epithelium of Apc fl/fl Kras fl/G12D mice but suppressed proliferation to a level below that of vehicle-treated Apc fl/fl Kras +/G12D mice (Fig. 4a ). We next tested whether MEK1/2 inhibition had a similar suppressive effect upon the process of intestinal tumourigenesis. To do this, we treated AKras fl/G12D or AKras +/G12D mice with AZD6244 (25mgkg -1 , BID) from 1-day post-induction of genetic recombination (Fig. 4b ). We found that inhibition of MEK1/2 had a modest impact on the survival of AKras +/G12D mice, based upon endpoint defined by onset of clinical signs associated with tumour burden, but significantly extended survival in AKras fl/G12D mice (median survival extended from 26 days to 115 days) (Fig. 4c ). This extension in survival was accompanied by a dramatic reduction in the number of small intestinal tumours (Fig. 4d ) alongside increase in colonic tumour number, albeit at greatly increased time post-induction. A significant reduction in tumour cell proliferation (BrdU incorporation) was also observed in AKras fl/G12D mice compared to AKras +/G12D derived tumours (Fig. 4e ). These data suggest that wild-type Kras acts to suppress the penetrance of mutant oncogenic Kras G12D , thus dampening MAPK signalling and contributing to therapeutic resistance in Kras mutant tumours, a key clinical problem. Fig. 4: Lack of wild-type Kras increases sensitivity to MEK inhibition in of KRASG12D colorectal tumours in vivo. a Left, quantification of BrdU-positive cells per half crypt in Apc fl/fl Kras +/G12D and Apc fl/fl Kras fl/G12D mice 3 days post-induction treated with Vehicle or MEKi (AZD6244) as indicated ( Apc fl/fl Kras +/G12D Vehicle, n = 5, 1M, 4F; MEKi, n = 4, 1M, 3F; and Apc fl/fl Kras fl/G12D Vehicle, n = 3, 1M, 2F; MEKi, n = 5, 3M, 2F). * P = 0.017. Right, representative H&E and BrdU images of Apc fl/fl Kras fl/G12D 3 days post-induction treated with Vehicle or MEKi (AZD6244) as indicated. Arrowheads show BrdU +ve hyper proliferative cells. Experiments carried out on C57BL/6J background ≥ N2. b Schematic presenting experimental approach. Apc +/fl Kras +/G12D and Apc +/fl Kras fl/G12D mice treated with MEKi one day post-induction and treated to clinical endpoint. Created with BioRender.com. c Kaplan–Meier survival curve of Apc +/fl Kras +/G12D and Apc +/fl Kras fl/G12D mice treated as shown in ( b ) aged until clinical endpoint ( Apc +/fl Kras +/G12D , n = 8, 2M, 6F, MS, median survival = 72; Apc +/fl Kras +/G12D MEKi, n = 6, 2M, 4F, MS, median survival = 96; Apc +/fl Kras fl/G12D , n = 4, 2M, 2F, MS, median survival = 22; Apc +/fl Kras fl/G12D MEKi, n = 5, 4M, 1F, MS, median survival = 115). ** P = 0.0050, ns not significant, log-rank (Mantel-Cox) test. d Boxplots showing total number of tumours from Apc +/fl Kras +/G12D and Apc +/fl Kras fl/G12D mice untreated or treated with MEKi as indicated in ( c ) and aged until clinical endpoint in SI and Colon ( Apc +/fl Kras +/G12D , n = 8, 2M, 6F; Apc +/fl Kras +/G12D MEKi, n = 5, 2M, 3F; Apc +/fl Kras fl/G12D , n = 4, 2M, 2F; Apc +/fl Kras fl/G12D MEKi, n = 5, 4M, 1F). ** P = 0.0079 ( Apc +/fl Kras fl/G12D SI), * P = 0.0281, * P = 0.0397 (colon). e Left: Representative BrdU images of Apc +/fl Kras +/G12D and Apc +/fl Kras fl/G12D tumours from mice treated with MEKi from day 1 post-induction until clinical endpoint. Right: boxplot showing percentage of BrdU-positive tumour cells in Apc +/fl Kras +/G12D and Apc +/fl Kras fl/G12D treated with MEKi ( Apc +/fl Kras +/G12D vehicle, n = 5, 1M, 2F; Apc +/fl Kras +/G12D MEKi, n = 5, 2M, 3F; Apc +/fl Kras fl/G12D untreated, n = 4, 2M, 2F; Apc +/fl Kras fl/G12D MEKi, n = 5, 4M, 1F), * P = 0.0159. a , d and e Boxes depict interquartile range, central line indicates median and whiskers indicate minimum/maximum values, one-way Mann–Whitney U test. Scale, 100 μm. Source data are provided as a Source Data file. Full size image Loss of wild-type KRAS potentiates oncogenic KRASG12D driven tumorigenesis in the absence of exogenous WNT mutations in vivo Within the intestinal epithelium KRAS mutation alone is not sufficient to drive tumourigenesis. Indeed, in human, KRAS mutant clones are known to commonly arise with age, in the intestinal epithelium in morphologically normal crypts. This is recapitulated by murine models where expression of an oncogenic Kras G12D mutant allele in isolation throughout the intestinal epithelium (villin-creERT2 Kras +/G12D ) results in lowly penetrant intestinal lesion development, which translates to an overall survival of greater than 12 months. Given the impact of combined deletion of wild-type Kras and expression of oncogenic Kras G12D on both intestinal homoeostasis, and tumour initiation in the context of heterozygous loss of Apc , we next asked whether these alterations in Kras allelic balance could drive tumour initiation in isolation. Here, we induced genetic recombination in villin-creERT2 Kras fl/G12D or villin-creERT2 Kras +/G12D mice, and assessed survival based upon sampling due to onset clinical signs associated with significant intestinal tumour burden. As expected, villin-creERT2 Kras +/G12D alone resulted in inefficient tumour initiation, with median survival for this group at around 16 months. Strikingly, mice in the villin-creERT2 Kras fl/G12D group developed tumours much more rapidly than the control group, exhibiting a greatly reduced median survival of around 230 days/9 months (Fig. 5a ). The tumours from both Kras fl/G12D and Kras +/G12D mice were predominantly found in the small intestine, and were characteristically large adenomas. However, tumour number was significantly increased in the small intestine of Kras fl/G12D mice (Fig. 5b, c ). This demonstrates that even when the only exogenously introduced driver mutation is Kras G12D , loss of wild-type Kras significantly promotes intestinal tumourigenesis, which in turn translates into significantly shortened survival. Fig. 5: Wild-type Kras deletion increases tumour initiation and alters progression of KRASG12D mutant colorectal tumours following loss of p53. a Kaplan–Meier survival curve of villin-creERT2 Kras +/G12D and Kras fl/G12D mice aged until clinical endpoint ( Kras +/G12D , n = 16, 5M, 11F; Kras fl/G12D , n = 12, 4M, 8F). **** P = 1.3 × 10 -9 . MS, median survival. b Dotplot showing total number of tumours from Kras +/G12D and Kras fl/G12D 2D mice. Data are mean ± s.e.m. ( Kras +/G12D , n = 11, 3M, 8F; Kras fl/G12D , n = 11, 4M, 7F). ** P = 0.0014. c Representative H&E and BrdU IHC images of Kras fl/G12D mice. Representative of 6 biological replicates per genotype. Dashed boxes highlight selected areas shown in high magnification. Scale, 200 µm. d Metacore Network analysis of differentially expressed genes from Kras fl/G12D tumours. e Geneset enrichment plot for Wnt beta-catenin signalling signature from the ‘Hallmark’ geneset collection of tumours derived from Kras fl/G12D mice. X -axis shows normalised enrichment score (NES), and the P value (computed and corrected for multiple testing using the Benjamini–Hochberg procedure). f Representative β-catenin IHC staining in Kras +/G12D and Kras fl/G12D mice. Representative of 5 biological replicates per genotype. Dashed boxes highlight selected areas shown in high magnification. Scale, 200 µm. g Kaplan–Meier survival curve of Kras +/G12D Trp53 fl/fl (KP) and Kras fl/G12D Trp53 fl/fl (KP KF) mice aged until clinical endpoint (KP, n = 10, 7M, 3F; KP KF, n = 16, 6M, 10F) **** P = 6 × 10 -8 . h Boxplots showing total number of tumours (left) and tumour burden, mm 2 (right) in KP and KP KF mice (KP, n = 7, 2M, 5F, KP KF, n = 15, 6M, 9F). * P = 0.02, ** P = 0.0017. Please note control KP cohort used in ( g ) and ( h ) comprise different mice. i Representative H&E, αSMA (alpha-smooth muscle actin) and Sirius Red staining of KP and KP KF tumours. Representative of KP n = 8; KP KF n = 5. Scale, 100 µm. j Boxplots showing Sirius Red positivity (%) and αSMA positive cells (%) of KP and KP KF tumours (KP n = 7; KP KF, n = 5). *P = 0.0326 (Sirius Red) , *P = 0.024 (αSMA). h and j boxes depict interquartile range, central line indicates median and whiskers indicate minimum/maximum values. P values in a and g are log-rank (Mantel-Cox) tests. b, h and j are one-way Mann–Whitney U tests. Source data are provided as a Source Data file. Full size image To better understand the mechanistic impact of deletion of wild-type Kras in the context of oncogenic Kras G12D , we transcriptionally profiled tumours arising in villin-creERT2 Kras fl/G12D mice and compared to adjacent non-transformed tissue. Geneset enrichment analysis (GSEA), identified key oncogenic programmes associated with KRAS signalling, MEK and AKT were enriched in villin-creERT2 Kras fl/G12D tumours (Supplementary Fig. 3a ). Importantly, GSEA and Metacore analysis of differentially expressed genes showed an overrepresentation of WNT and β-catenin signalling pathways (Fig. 5d, e ). Given that aberrant activation of the Wnt/β-catenin pathway, and its downstream transcriptional networks, is a common initiating event in CRC, and results from stabilisation and nuclear accumulation of the transcriptional co-activator β-catenin, we interrogated tumours arising in villin-creERT2 Kras fl/G12D and villin-creERT2 Kras +/G12D mice for nuclear accumulation of β-catenin. Consistent with the transcriptional enrichment of Wnt signalling pathways (Fig. 5e ), tumours arising in Kras fl/G12D intestines showed positivity for nuclear β-catenin while Kras +/G12D intestines more predominantly exhibited membranous β-catenin (Fig. 5f ). Loss of wild-type KRAS alters tumour progression and metastasis of aggressive mutant KRAS-driven colorectal tumours Thus far, we have only investigated the role of wild-type KRAS in mouse models of adenoma. Recent reports have shown that changes in KRAS gene dosage alter the clonal evolution of tumours and change the metastatic incidence in KRAS mutant cancers [23] . Given the dramatic role we have observed in tumour initiation, we next wished to see how important wild-type KRAS would be in tumour progression. We have previously demonstrated that deletion or mutation of the tumour suppressor gene Trp53 alongside activating mutation of Kras can give rise to aggressive, late-stage adenocarcinoma development in the intestine [32] . Indeed, the human paralogue, TP53 is inactivated in more than half of human colorectal cancers (TCGA). These models therefore represent an ideal system for interrogating the impact of wild-type Kras deletion in a more complex, aggressive, clinically relevant oncogenic KRAS G12D driven disease. 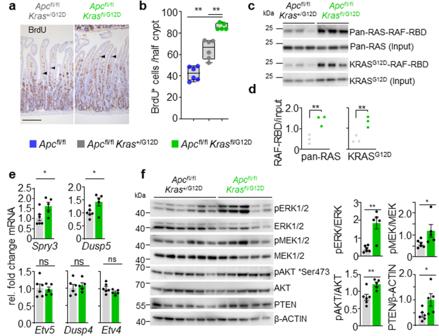Fig. 2: Wild-typeKrasdeletion increases proliferation, active KRAS and MAPK signalling. aRepresentative H&E and BrdU IHC ofApcfl/flKras+/G12DandApcfl/flKrasfl/G12Dmice sampled 3 days post Cre-induction. Arrowheads indicate de-differentiating cells in the villi. Scale, 100 μm.bBoxplots showing BrdU-positive cells from at least 25 half-crypts in SI inApcfl/fl, Apcfl/flKras+/G12DandApcfl/flKrasfl/G12Dmice. Boxes depict interquartile range, central line indicates median and whiskers indicate minimum/maximum values(Apcfl/fl,n=6, 4M, 2F; Apcfl/flKras+/G12D,n= 6, 2M, 4F; andApcfl/flKrasfl/G12D,n= 5, 1M, 4F mice). **P= 0.0022, **P= 0.0043.cRAF-Ras Binding Domain (RBD) agarose affinity purification assay of three biologically independent samples per condition fromApcfl/flKras+/G12Dand Apcfl/flKrasfl/G12Dintestinal organoids. Pulldown of RAS-GTP with RAF-RBD agarose beads. Top: Precipitates were immunoblotted using a pan-RAS antibody and input pan-RAS served as loading control. RAS-GTP activation levels were quantified and normalised to pan-Ras loading control.Apcfl/flKras+/G12D,n= 3, 2M, 1F; andApcfl/flKrasfl/G12D,n= 3, 1M, 2F. Bottom: Precipitates were immunoblotted using a KRASG12D antibody and input KRASG12D served as loading control. KRASG12D-RAF-RBD levels were quantified and normalised to KRASG12D loading control.Apcfl/flKras+/G12D,n= 3, 3M; andApcfl/flKrasfl/G12D,n= 3, 1M, 2F.dQuantification of RAF-RBD assay (left) and KRASG12D immunoblot (right fromc), **P= 0.0045 (pan-RAS), **P= 0.0044 (KRASG12D).eqRT-PCR analysis ofEtv5, Etv4, Dusp4, Dusp5andSpry3inApcfl/flKras+/G12D(n= 6, 3M, 3F) andApcfl/flKrasfl/G12D(n= 5, 1M, 4F) intestinal organoids. Data are mean ± s.e.m. Transcript levels were normalised toGapdh. *P= 0.0260 (Spry3) *P= 0.0411 (Dusp5).fLeft: Immunoblots showing PTEN, pAKT (Ser473), AKT, pERK1/2, ERK1/2, pMEK1/2, MEK1/2 and ß-actin inApcfl/flKras+/G12Dand Apcfl/flKrasfl/G12Dintestinal organoids. 6Apcfl/flKras+/G12Dand5Apcfl/flKrasfl/G12Dbiological replicates per group, each lane represents organoids generated from individual mice from genotype indicated. Right: Quantification of immunoblots, phosphorylated proteins were normalised to total protein levels. Data are mean ± s.e.m. **P= 0.0043 (pERK/ERK), *P= 0.0152 (pMEK/MEK), **P= 0.0087 (pAKT/AKT), *P= 0.015 (PTEN/ß-actin).b,d,e,fusing one-way Mann–WhitneyUtest. Source data are provided as a Source Data file. To achieve this, we interbred the villin-creERT2 Kras fl/G12D mouse line with a Trp53 conditional knockout allele to generate villin-creERT2 Kras fl/G12D Trp53 fl/fl (henceforth referred to as KP KF) and villin-creERT2 Kras +/G12D Trp53 fl/fl (henceforth referred to as KP) mice. While KP mice developed on average one intestinal tumour and exhibited a median overall survival of 240 days, with very lowly penetrant metastasis (Fig. 5g, h ), KP KF mice developed on average four intestinal tumours and exhibited a median overall survival of 150 days (Fig. 5g, h ). Histological analysis of tumours arising in KP KF mice suggested a morphology akin to human tubulovillous adenoma, in contrast to the tumours which arose in control KP mice, which exhibit a serrated morphology. Moreover, evidence of local invasion or poor differentiation, features typically associated with advanced disease, were apparent in KP tumours but absent from KP KF tumours (Fig. 5i ). In addition, there were clear differences in the stromal microenvironment of the KP KF tumours, such as a lack of infiltrating alpha-smooth muscle actin (αSMA)-positive stromal cells and low levels of stromal collagen deposition (as indicated by picrosirius red), again, contrasted by KP tumours (Fig. 5i, j ). These data suggest that while loss of the wild-type copy of Kras in an aggressive Kras mutant-driven model of intestinal cancer can drive accelerated tumour initiation, it does not endow tumours with increased invasion or aggression, indeed these features appear suppressed. Considering this, we decided to further investigate the role of wild-type Kras in aggressive, late-stage KRAS-mutant CRC using our recently described metastatic KPN model (villin-creERT2 Kras +/G12D Trp53 fl/fl Rosa26 N1icd/+ ). These KPN mice develop intestinal adenocarcinoma and exhibit highly penetrant metastasis, predominantly to the liver [32] . We interbred KPN mice with KP KF mice to generate (villin-creERT2 Kras fl/G12D Trp53 fl/fl Rosa26 N1icd/+ ; henceforth referred to as KPN KF). Strikingly, tumorigenesis was significantly accelerated in KPN KF mice with deletion of wild-type Kras , reflected by a significant reduction in overall survival based upon endpoint defined by clinical signs associated with tumour burden (Fig. 6a ). Using droplet PCR we confirmed this acceleration in tumorigenesis of KPN KF mice was not due to mutant Kras induced changes in Kras copy number (Supplementary Fig. 4a, b ). Comparative histological analysis of tumours from KPN and KPN KF mice showed that tumours arising from KPN KF showed lack of local invasion with remarkable lack of metastasis incidence (Fig. 6b, c ). To gain a better mechanistic insight into the impact of Kras deletion in this setting, we first performed transcriptional analysis of tumours derived from KPN KF and KPN mice. Interestingly, KPN KF tumours showed a significant enrichment of Wnt signalling pathway (Fig. 6d ) and expression of the surrogate Wnt marker Notum , compared to KPN tumours (Fig. 6e, f ). It is notable that relatively low levels of Wnt activation is a key feature of the highly metastatic KPN tumours, while comparable high-Wnt APC-deficient, APN tumours are non-metastatic [32] . Consistent with the high-Wnt activation signature in KPN KF tumours, comparative analysis of several published Wnt transcriptional signatures in tumours from APN, KPN and KPN KF mice clearly showed higher Wnt activation in KPN KF tumours (Supplementary Fig. 4c ). Collectively, these data show that Kras mutant tumours lacking wild-type Kras in a KPN setting activate more robust levels of Wnt signalling during tumorigenesis. This said, it is noteworthy that primary tumours arising in the intestine of KPN KF mice are adenomatous, while those arising in KPN mice are of a more aggressive adenocarcinoma/carcinomatous morphology. While the underlying genetics will undoubtedly play a key role in defining the molecular makeup of the disease, the reduced histopathological grade of tumours found in KPN KF may directly influence immune and inflammatory infiltrate. Fig. 6: Wild-type Kras deletion alters progression and metastasis of KPN tumours. a Kaplan–Meier survival curve of Kras +/G12D Trp53 fl/fl Rosa26 N1icd/+ (KPN) and Kras fl/G12D Trp53 fl/fl Rosa26 N1icd/+ (KPN KF) mice aged until clinical endpoint (KPN, n = 10, 5M, 5F, KPN KF, n = 12, 6M, 6F) *** P = 2 × 10 -4, log-rank (Mantel-Cox) test. b Representative H&E images of primary tumour and metastasis (liver) of mice from ( a ). Scale, 200 μm. c Incidence of metastasis (%) in KPN and KPN KF mice aged until clinical endpoint (KPN, n = 11, 6M, 5F; KPN KF, n = 11, 5M, 6F) **** P = 1 × 10 -15, two-tailed chi-square test. d GSEA of hallmark WNT-β-Catenin signalling in KPN KF tumours compared to KPN. X -axis shows normalised enrichment score (NES), and the P value (computed and corrected for multiple testing using the Benjamini–Hochberg procedure). e Representative Notum in situ hybridisation (ISH) in KPN and KPN KF tumours. Scale, 100 μm. f Boxplots showing Notum (ISH) positive cells per tumour (%) of KPN and KPN KF tumours (KPN, n = 7, 2M, 5F; KPN KF, n = 5, 2M, 3F). **P = 0.0013. g Dotplot showing neutrophils percentage in systemic blood of KPN and KPN KF mice aged to clinical endpoint (KPN, n = 8, 6M, 2F; KPN KF, n = 7, 5M, 2F). *** P = 0.0006. h Representative Cxcl5 ISH in KPN and KPN KF tumours. Representative of five mice per genotype. Scale, 100 μm. i Boxplots showing Cxcl5 positive cells per tumour (%) of KPN and KPN KF tumours (KPN, n = 6, 2M, 4F; KPN KF, n = 5, 2M, 3F). *P = 0.0411. j Volcano plot of differentially expressed genes in organoids derived from KPN KF tumours. k Relative expression of Tgfβ ligands and chemokines from organoids derived from KPN and KPN KF tumours. Data are mean ± s.e.m. KPN, n = 3, 3M; KPN KF, n = 4, 1M, 3F. l Representative αSMA (alpha-smooth muscle actin) and Sirius Red staining of KPN and KPN KF tumours. Scale, 200 µm. m Boxplots showing Sirius Red positivity (%) and αSMA positive cells (%) of ageing or vehicle-treated KPN and KPN KF tumours (KPN n = 7, 2M, 5F; KPN KF n = 8, 4M, 4F). *P = 0.0103. f , i and m boxes depict interquartile range, central line indicates median and whiskers indicate minimum/maximum values. f , g , i and m are one-way Mann–Whitney U tests. Source data are provided as a Source Data file. Full size image Nonetheless, we have previously shown that a critical feature of metastasis in the Notch1-driven KPN tumours is TGFβ pathway-mediated neutrophil infiltration [32] . However, we detected a lack of systemic circulating neutrophil accumulation in the blood of KPN KF mice (Fig. 6g ). Given that chemokines such as Cxcl5 are implicated in neutrophil attraction, we assessed expression of Cxcl5 and found significantly reduced expression in the epithelium of KPN KF tumours (Fig. 6h, i ). 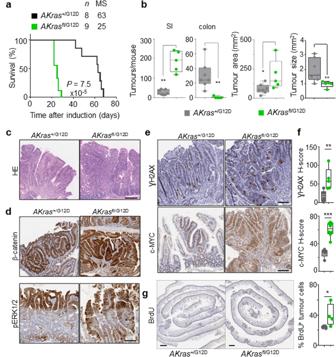Fig. 3: Loss of wild-typeKrasincreases mutant KRAS-driven tumourigenesis together withApcloss. aKaplan–Meier survival curve of villin-creERT2Apc+/flKras+/G12D(AKras+/G12D) and villin-creERT2Apc+/flKrasfl/G12D(AKrasfl/G12D) mice aged until clinical endpoint (Apc+/flKras+/G12D,n= 8, 5M, 3F, MS, median survival = 63;Apc+/flKrasfl/G12D,n= 9, 5M, 4F, MS, median survival = 25), ****P= 7.5 × 10-5, log-rank (Mantel-Cox) test.bLeft: Boxplots showing total number of tumours fromApc+/flKras+/G12DandApc+/flKrasfl/G12Dmice aged until clinical endpoint in SI and Colon. Right: Boxplots showing tumour area (mm2) and tumour size (mm2) inApc+/flKras+/G12DandApc+/flKrasfl/G12Dmice aged until clinical endpoint. Boxes depict interquartile range, central line indicates median and whiskers indicate minimum/maximum values (Apc+/flKras+/G12D,n= 7, 5M, 2F;Apc+/flKrasfl/G12Dn= 5, 3M, 2F). **P= 0.0013 (SI), **P= 0.0013 (colon), *P= 0.036 (area), **P= 0.0088 (size), one-way Mann–WhitneyUtest.cRepresentative H&E images ofAKras+/G12D(n= 5, 2M, 3F) andAKrasfl/G12D(n= 8, 5M, 3F) tumour. Dashed box highlights selected area shown in high magnification.dRepresentative images of nuclear β-catenin and pERK1/2 staining inApc+/flKras+/G12D(n= 5, 2M, 3F) andApc+/flKrasfl/G12D(n= 8, 5M, 3F) tumours at clinical endpoint. Scale, 100 µm.eRepresentative images of γH2AX and c-MYC staining inApc+/flKras+/G12D(n= 5, 2M, 3F) andApc+/flKrasfl/G12D(n= 8, 5M, 3F) tumours at clinical endpoint. Scale, 100 µm.fH-score of γH2AX (Apc+/flKras+/G12D,n= 6, 4M, 2F;Apc+/flKrasfl/G12Dn= 5, 3M, 2F) and c-MYC (Apc+/flKras+/G12D,n= 5, 2M, 3F;Apc+/flKrasfl/G12Dn= 8, 5M, 3F) IHC staining of (e). Boxes depict interquartile range, central line indicates median and whiskers indicate minimum/maximum values. **P= 0.0043, ***P= 0.0008, one-way Mann–WhitneyUtest.gRepresentative BrdU staining ofApc+/flKras+/G12DandApc+/flKrasfl/G12Dsmall intestinal tumours at clinical endpoint. Scale, 100 µm. Right: quantification of BrdU positivity in tumour cells. Boxes depict interquartile range, central line indicates median and whiskers indicate minimum/maximum values. (Apc+/flKras+/G12D,n= 5, 3M, 2F;Apc+/flKrasfl/G12Dn= 4, 2M, 2F). *P=0.0317, one-way Mann–WhitneyUtest. Source data are provided as a Source Data file. To determine how loss of wild-type Kras alters the TGFβ pathway and metastasis, we examined the transcriptome of tumour-derived KPN and KPN KF organoids. Interestingly, we found that NOTCH1-mediated gene expression of Tgfb2 and chemokines, such as Cxcl1, Cxcl3 and Cxcl5 , was downregulated in KPN KF organoids (Fig. 6j, k ). Moreover, GSEA analysis showed lack of TGFβ signalling in KPN KF organoids (Supplementary Fig. 4d ). Furthermore, along with the low expression of neutrophil markers (Fig. 6h, i ), Tgfb2 expression was lowered in KPN KF tumours (Supplementary Fig. 4e ). In addition, we observed clear differences in the stromal microenvironment of the KPN KF tumours, with significantly low stromal collagen deposition (picrosirius red), again, contrasted by collagen high KPN tumours (Fig. 6l, m ). Given that we have previously shown that KPN tumour cells generate an immunosuppressive, pro-metastatic environment, we assessed the ability of KPN KF tumour cells to produce such an immunosuppressive environment to generate distant metastasis. To address this experimentally, we performed orthotopic intrasplenic transplantation of KPN and KPN KF tumour-derived organoids in syngeneic recipient mice (Fig. 7a ). All mice with KPN organoid transplantation showed metastasis to either liver or lung (Fig. 7b ). However, the metastasis burden was significantly blunted in KPN KF organoid transplanted mice (Fig. 7b, c ). Remarkably, we saw a significant increase in immune cell infiltration in KPN KF transplants compared to the KPN control tumours (Fig. 7d, e ). The observed impact upon immune and inflammatory infiltrate was independent of the size of metastatic deposits found in the liver – the decreased neutrophil and increased lymphocyte association with metastatic deposits in KPN KF transplants versus KPN transplants was maintained when analysis was restricted to tumours of comparable size (Supplementary Fig. 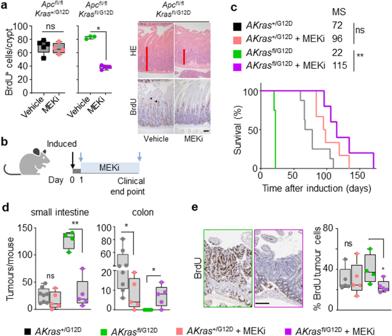Fig. 4: Lack of wild-typeKrasincreases sensitivity to MEK inhibition in of KRASG12D colorectal tumours in vivo. aLeft, quantification of BrdU-positive cells per half crypt inApcfl/flKras+/G12DandApcfl/flKrasfl/G12Dmice 3 days post-induction treated with Vehicle or MEKi (AZD6244) as indicated (Apcfl/flKras+/G12DVehicle,n= 5, 1M, 4F; MEKi,n= 4, 1M, 3F; andApcfl/flKrasfl/G12DVehicle,n= 3, 1M, 2F; MEKi,n= 5, 3M, 2F). *P= 0.017. Right, representative H&E and BrdU images ofApcfl/flKrasfl/G12D3 days post-induction treated with Vehicle or MEKi (AZD6244) as indicated. Arrowheads show BrdU+vehyper proliferative cells. Experiments carried out on C57BL/6J background ≥ N2.bSchematic presenting experimental approach.Apc+/flKras+/G12DandApc+/flKrasfl/G12Dmice treated with MEKi one day post-induction and treated to clinical endpoint. Created with BioRender.com.cKaplan–Meier survival curve ofApc+/flKras+/G12DandApc+/flKrasfl/G12Dmice treated as shown in (b) aged until clinical endpoint (Apc+/flKras+/G12D,n= 8, 2M, 6F, MS, median survival = 72;Apc+/flKras+/G12DMEKi,n= 6, 2M, 4F, MS, median survival = 96;Apc+/flKrasfl/G12D,n= 4, 2M, 2F, MS, median survival = 22;Apc+/flKrasfl/G12DMEKi,n= 5, 4M, 1F, MS, median survival = 115). **P= 0.0050, ns not significant, log-rank (Mantel-Cox) test.dBoxplots showing total number of tumours fromApc+/flKras+/G12DandApc+/flKrasfl/G12Dmice untreated or treated with MEKi as indicated in (c) and aged until clinical endpoint in SI and Colon (Apc+/flKras+/G12D,n= 8, 2M, 6F;Apc+/flKras+/G12DMEKi,n= 5, 2M, 3F;Apc+/flKrasfl/G12D,n= 4, 2M, 2F;Apc+/flKrasfl/G12DMEKi,n= 5, 4M, 1F). **P= 0.0079 (Apc+/flKrasfl/G12DSI), *P= 0.0281, *P= 0.0397 (colon).eLeft: Representative BrdU images ofApc+/flKras+/G12DandApc+/flKrasfl/G12Dtumours from mice treated with MEKi from day 1 post-induction until clinical endpoint. Right: boxplot showing percentage of BrdU-positive tumour cells inApc+/flKras+/G12DandApc+/flKrasfl/G12Dtreated with MEKi (Apc+/flKras+/G12Dvehicle,n= 5, 1M, 2F;Apc+/flKras+/G12DMEKi,n= 5, 2M, 3F;Apc+/flKrasfl/G12Duntreated,n= 4, 2M, 2F;Apc+/flKrasfl/G12DMEKi,n= 5, 4M, 1F), *P= 0.0159.a,dandeBoxes depict interquartile range, central line indicates median and whiskers indicate minimum/maximum values, one-way Mann–WhitneyUtest. Scale, 100 μm. Source data are provided as a Source Data file. 5a, b ). Moreover, the apparent impact upon immune cell infiltration was also confirmed in the KPN KF GEMM tumours (Supplementary Fig. 4g ). Together, this indicates that loss of wild-type Kras with epithelial NOTCH1 activation in KPN tumours activates Wnt, restricts the TGFβ mediated neutrophil recruitment required to generate an immunosuppressive, pro-metastatic niche and blunts the metastases of tumours lacking wild-type Kras (Fig. 7f ). Fig. 7: Wild-type Kras deficient KPN cells show reduced metastatic capacity and increased immune infiltration. a Schematic showing the intrasplenic transplantation of KPN and KPN KF organoids. b Images of liver tumour burden from KPN and KPN KF organoid transplant mice. Representative of six mice per organoid transplant. Scale, 1 cm. c Quantifications of liver tumour burden and tumour number from KPN and two KPN KF (T1 and T2) organoid transplants. (KPN n = 6, 6M, KPN KF T1 n = 7, 7F, KPN KF T2 n = 7, 7F). Data are mean ± s.e.m. Semi-circles include lung metastasis burden. ***P = 0.0006, one-way Mann–Whitney U test. Created with BioRender.com. d Representative HE, CD3, CD8, F4/80 and S100A9 IHC in KPN and KPN KF transplant mice. Representative of six mice per organoid line. Scale, 200 μm. e Quantifications from d KPN KF T1 and T2 with tumour burden represented together as KPN KF. Data are mean ± s.e.m. Representative of KPN n = 6, 6M, KPN KF n = 14, 14F, ****P = 2.5 × 10 -5 (Met area); KPN n = 5, 5M, KPN KF n = 7, 7F, **P = 0.0013 (CD3); KPN n = 5, 5M, KPN KF n = 6, 6F, ns, P = 0.2143 (CD8); KPN n = 6, 6M, KPN KF n = 5, 5F, *P = 0.02 (F4/80); KPN n = 5, 5M, KPN KF n = 5, 5F, **P = 0.0079 (S100A9), one-way Mann–Whitney U test. f Schematic model showing the role of wild-type KRAS in KRAS mutant CRC. Loss of wild-type Kras in KPN KF tumours promotes tumour initiation with WNT activation, an enhanced immune infiltrate and blunted metastasis. Created with BioRender.com. Source data are provided as a Source Data file. Full size image 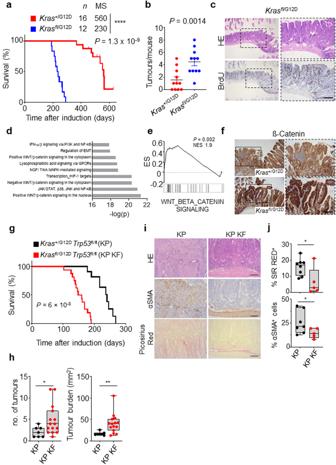Fig. 5: Wild-typeKrasdeletion increases tumour initiation and alters progression of KRASG12D mutant colorectal tumours following loss of p53. aKaplan–Meier survival curve of villin-creERT2Kras+/G12DandKrasfl/G12Dmice aged until clinical endpoint (Kras+/G12D,n= 16, 5M, 11F;Krasfl/G12D,n= 12, 4M, 8F). ****P= 1.3 × 10-9. MS, median survival.bDotplot showing total number of tumours fromKras+/G12DandKrasfl/G12D2D mice. Data are mean ± s.e.m. (Kras+/G12D,n= 11, 3M, 8F;Krasfl/G12D,n= 11, 4M, 7F). **P= 0.0014.cRepresentative H&E and BrdU IHC images ofKrasfl/G12Dmice. Representative of 6 biological replicates per genotype. Dashed boxes highlight selected areas shown in high magnification. Scale, 200 µm.dMetacore Network analysis of differentially expressed genes fromKrasfl/G12Dtumours.eGeneset enrichment plot for Wnt beta-catenin signalling signature from the ‘Hallmark’ geneset collection of tumours derived fromKrasfl/G12Dmice.X-axis shows normalised enrichment score (NES), and thePvalue (computed and corrected for multiple testing using the Benjamini–Hochberg procedure).fRepresentative β-catenin IHC staining inKras+/G12DandKrasfl/G12Dmice. Representative of 5 biological replicates per genotype. Dashed boxes highlight selected areas shown in high magnification. Scale, 200 µm.gKaplan–Meier survival curve ofKras+/G12DTrp53fl/fl(KP) andKrasfl/G12DTrp53fl/fl(KP KF) mice aged until clinical endpoint (KP,n= 10, 7M, 3F; KP KF,n= 16, 6M, 10F) ****P= 6 × 10-8.hBoxplots showing total number of tumours (left) and tumour burden, mm2(right) in KP and KP KF mice (KP,n= 7, 2M, 5F, KP KF,n= 15, 6M, 9F). *P= 0.02, **P= 0.0017. Please note control KP cohort used in (g) and (h) comprise different mice.iRepresentative H&E, αSMA (alpha-smooth muscle actin) and Sirius Red staining of KP and KP KF tumours. Representative of KPn= 8; KP KFn= 5. Scale, 100 µm.jBoxplots showing Sirius Red positivity (%) and αSMA positive cells (%) of KP and KP KF tumours (KPn= 7; KP KF,n= 5).*P= 0.0326 (Sirius Red), *P=0.024 (αSMA).handjboxesdepict interquartile range, central line indicates median and whiskers indicate minimum/maximum values.Pvalues inaandgare log-rank (Mantel-Cox) tests.b, handjare one-way Mann–Whitney U tests. Source data are provided as a Source Data file. Activating mutations in proto-oncogenes like KRAS are the initial events in the development of cancer followed by sequential progression involving additional genetic hits in tumour suppressor genes. Here we provide evidence that loss of wild-type Kras facilitates and accelerates tumour initiation, but drastically alters tumour evolution in CRC. We demonstrate that loss of wild-type Kras increases the dependence of these tumours on the MAPK pathway thereby making them susceptible for targeting through MEK1/2 inhibition. In addition, we find that loss of tumour suppressors like p53 together with loss of wild-type Kras leads to faster tumour initiation but altered progression in Kras mutant tumours. The role of wild-type RAS isoforms is contradictory in tumours. While the biochemical properties and transforming potential of RAS oncoproteins suggest a dominant mechanism for these mutant proteins during tumorigenesis, several studies have argued for and against the antagonising properties of wild-type RAS in the presence of oncogenic variants [18] , [33] , [34] . There is also evidence that this is context dependent based on the RAS isoform and the tissue type under investigation [35] . Early reports suggested that presence of wild-type Hras or Nras can suppress tumourigenic phenotypes of mutant RAS encoding genes [36] . While loss of wild-type Kras was shown to promote activation of all RAS isoforms in a leukaemia model [37] , loss of wild-type Nras did not alter the tumorigenic behaviour of mutant NRAS-G12D in a hematopoietic cancer model [38] . Our genetic and functional analyses using Kras mutant mouse models of colorectal cancer suggest that wild-type Kras plays a significant role in the cancer cell fitness, evolution and therapeutic susceptibility of Kras mutant cells in vivo. Recent reports have highlighted that not all KRAS mutations are equal, with each KRAS mutation having unique biochemical, signalling and functional properties in cells [5] , [6] , [7] . Our data suggest that these well-characterised isoform-specific differences may be further compounded by allelic changes such as loss of the wild-type allele. Recent work from Ambrogio et al. suggested that dimerization of oncogenic KRAS is essential to sustain oncogenic function and the growth inhibitory effect of wild-type KRAS is linked to its dimerization with mutant KRAS [19] . We show that wild-type Kras suppresses phenotypes associated with mutant Kras in colorectal models in vivo. While KRAS-driven CRC and PDAC are resistant to MEKi, the KRAS allelic configuration has been shown to modulate MEKi sensitivity in AML and CRC cell lines [1] . Our data show that loss of wild-type Kras causes cancer cells to amplify oncogenic signalling to optimise growth, leading them to be more dependent or addicted to certain activated pathways that become therapeutic susceptibilities. The enhanced sensitivity of Kras G12D/fl tumours to MEKi supports this idea. Similarly, this would also suggest that in addition to screening of patients for KRAS mutation status, stratification of patients with KRAS allelic status that corresponds to selective pressure for outgrowth of tumours with increased MAPK signalling are more likely to render this subset of patients more susceptible to effector pathway inhibitors. The idea that mutant KRAS gene dosage or allelic configuration can alter tumour progression has been explored recently. It is notable that as such changes are reported to be common and occur in high frequencies in KRAS mutant cancers, our data argue that loss of wild-type Kras significantly increases initiation of Kras mutant intestinal tumours [23] , [26] . In contrast to Kras +/G12D tumours, we find that Kras fl/G12D tumours exhibit a reduction in serration, alongside reduced invasion, differentiation, and metastasis – all features previously associated with high levels of Wnt signalling in CRC. We have previously identified TGFB2 and other chemokine secretion from the epithelium, driven by Notch activation as a key driver of metastasis in mouse models of CRC [32] . Considering the co-ordinated control of, and commonly reciprocal relationship between Wnt and Notch signalling in CRC [39] , it is intriguing that the suppression of metastasis observed in complex Kras fl/G12D tumours occurs hand-in-hand with transcriptional enrichment of canonical Wnt-associated gene programmes. This is also consistent with reports showing that Wnt-high human CRC with elevated expression of Wnt target genes have better prognosis than Wnt-low tumours [40] , [41] . In the model systems reported here, Wnt-dependent transcriptional programmes were enriched in Kras fl/G12D tumours when compared to Kras +/G12D intestinal tumours, indicative of further crosstalk between the Kras and Wnt signalling pathways. When viewed in the round, these observations suggest complex interplay between the WNT, NOTCH and KRAS signalling axes in determining disease trajectory in colorectal cancer, and that allelic imbalances at the KRAS locus might skew this relationship, ultimately impacting prognosis and therapeutic sensitivity. Mouse models and experiments All experiments were performed according to UK Home Office regulations (Project licences 70/8646, PP3908577), under the oversight of the Animal Welfare and Ethical Review Board (AWERB) of the University of Glasgow. Mice were genotyped by Transnetyx (Cordoba, TN, USA). For all experiments, male and female mice of >20 g and between 6 and 15 weeks of age were used, unless otherwise specified. For intestinal studies, the transgenes and alleles used were as follows – villin-creERT2 [42] , Apc fl [43] , Kras LSL-G12D [44] , Braf V600E(tm1Mmcm) [45] , Braf V600E(tm1Cpri) [46] , Trp53 fl [47] and Rosa26 N1icd [48] . Recombination by Villin-creERT2 was induced with one intraperitoneal (i.p.) injection of 80 mg/kg tamoxifen on day 0. Analysis of villin-creERT2-induced Apc fl/fl Kras +/G12D and Apc fl/fl Kras fl/G12D mice was at day 3 after induction. For tumourigenesis studies, villin-creERT2 Apc +/fl (with Kras +/G12D or Kras fl/G12D ), Kras +/G12D , Kras fl/G12D , KP, KP KF, KPN and KPN KF mice were sampled when exhibiting clinical signs of ill-health indicative of substantial intestinal tumour burden (typically anaemia, hunching and/or weight loss), with overall survival recorded as the time from induction to sampling. Mice and organoids comprising the were of a C57BL/6J background, backcrossed ≥ 6 generations, unless otherwise stated. The MEK inhibitor (AZD6244 or selumetinib) was administered in a concentration of 25 mg/kg twice daily via oral gavage in a vehicle of 0.5% HPMC and 0.1% Tween-80. Intrasplenic transplantation injections were performed as previously described [32] using a cell suspension of primary tumour organoids derived from C57BL/6 KPN or KPN KF mice. Organoid donor and recipient mice were strain matched. Metastatic tumour burden and tumour number were scored macroscopically upon dissection, with tumour burden recorded as cumulative area of metastatic deposit observed across all liver lobules from each individual mouse. For analysis of composition of size-matched metastatic deposits, the mean area of metastatic deposit from the KPN KF cohort was calculated microscopically from a single H&E liver section per mouse. This value ± 1 × standard deviation (σ) was used as a range of tumour area (21188.95–154971.4 µm 2 ), which could in turn be used to select size-matched metastatic deposits from the KPN cohort for comparative analysis. 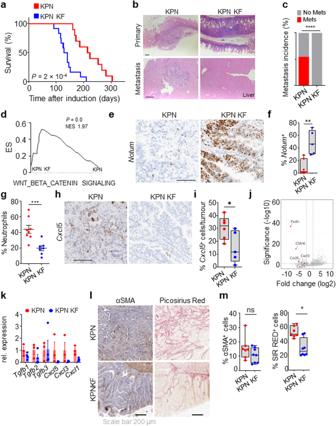Fig. 6: Wild-typeKrasdeletion alters progression and metastasis of KPN tumours. aKaplan–Meier survival curve ofKras+/G12DTrp53fl/flRosa26N1icd/+(KPN) andKrasfl/G12DTrp53fl/flRosa26N1icd/+(KPN KF) mice aged until clinical endpoint (KPN,n= 10, 5M, 5F, KPN KF,n= 12, 6M, 6F) ***P= 2 × 10-4,log-rank (Mantel-Cox) test.bRepresentative H&E images of primary tumour and metastasis (liver) of mice from (a). Scale, 200 μm.cIncidence of metastasis (%) in KPN and KPN KF mice aged until clinical endpoint (KPN,n= 11, 6M, 5F; KPN KF,n= 11, 5M, 6F) ****P= 1 × 10-15,two-tailed chi-square test.dGSEA of hallmark WNT-β-Catenin signalling in KPN KF tumours compared to KPN.X-axis shows normalised enrichment score (NES), and thePvalue (computed and corrected for multiple testing using the Benjamini–Hochberg procedure).eRepresentativeNotumin situ hybridisation (ISH) in KPN and KPN KF tumours. Scale, 100 μm.fBoxplots showingNotum(ISH) positive cells per tumour (%) of KPN and KPN KF tumours (KPN,n= 7, 2M, 5F; KPN KF,n= 5, 2M, 3F).**P= 0.0013.gDotplot showing neutrophils percentage in systemic blood of KPN and KPN KF mice aged to clinical endpoint (KPN,n= 8, 6M, 2F; KPN KF,n= 7, 5M, 2F). ***P= 0.0006.hRepresentativeCxcl5ISH in KPN and KPN KF tumours. Representative of five mice per genotype. Scale, 100 μm.iBoxplots showingCxcl5positive cells per tumour (%) of KPN and KPN KF tumours (KPN,n= 6, 2M, 4F; KPN KF,n= 5, 2M, 3F).*P= 0.0411.jVolcano plot of differentially expressed genes in organoids derived from KPN KF tumours.kRelative expression ofTgfβligands and chemokines from organoids derived from KPN and KPN KF tumours. Data are mean ± s.e.m. KPN,n= 3, 3M; KPN KF,n= 4, 1M, 3F.lRepresentative αSMA (alpha-smooth muscle actin) and Sirius Red staining of KPN and KPN KF tumours. Scale, 200 µm.mBoxplots showing Sirius Red positivity (%) and αSMA positive cells (%) of ageing or vehicle-treated KPN and KPN KF tumours (KPNn= 7, 2M, 5F; KPN KFn= 8, 4M, 4F).*P=0.0103.f,iandmboxes depict interquartile range, central line indicates median and whiskers indicate minimum/maximum values.f,g,iandmare one-way Mann–WhitneyUtests. Source data are provided as a Source Data file. 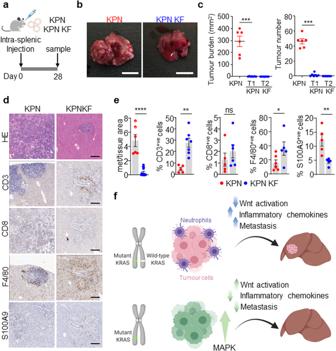Fig. 7: Wild-typeKrasdeficient KPN cells show reduced metastatic capacity and increased immune infiltration. aSchematic showing the intrasplenic transplantation of KPN and KPN KF organoids.bImages of liver tumour burden from KPN and KPN KF organoid transplant mice. Representative of six mice per organoid transplant. Scale, 1 cm.cQuantifications of liver tumour burden and tumour number from KPN and two KPN KF (T1 and T2) organoid transplants. (KPNn= 6, 6M, KPN KF T1n= 7, 7F, KPN KF T2n= 7, 7F). Data are mean ± s.e.m. Semi-circles include lung metastasis burden.***P= 0.0006, one-way Mann–WhitneyUtest. Created with BioRender.com.dRepresentative HE, CD3, CD8, F4/80 and S100A9 IHC in KPN and KPN KF transplant mice. Representative of six mice per organoid line. Scale, 200 μm.eQuantifications fromdKPN KF T1 and T2 with tumour burden represented together as KPN KF. Data are mean ± s.e.m. Representative of KPNn= 6, 6M, KPN KFn= 14, 14F,****P= 2.5 × 10-5(Met area); KPNn= 5, 5M, KPN KFn= 7, 7F,**P= 0.0013 (CD3); KPNn= 5, 5M, KPN KFn= 6, 6F, ns,P= 0.2143 (CD8); KPNn= 6, 6M, KPN KFn= 5, 5F,*P= 0.02 (F4/80); KPNn= 5, 5M, KPN KFn= 5, 5F,**P= 0.0079 (S100A9), one-way Mann–WhitneyUtest.fSchematic model showing the role of wild-type KRAS in KRAS mutant CRC. Loss of wild-typeKrasin KPN KF tumours promotes tumour initiation with WNT activation, an enhanced immune infiltrate and blunted metastasis. Created with BioRender.com. Source data are provided as a Source Data file. The smallest sample size was chosen that could give a significant difference, in accordance with the 3Rs. Given the robust phenotypes of the villin-creERT2 Apc fl/fl model, and prediction that KRAS was essential, the minimum size sample size assuming no overlap in control vs. experimental is three animals. Generation of Kras and Braf conditional alleles To generate conditional alleles of Kras and Braf , embryonic stem cell lines (mESCs) were imported from EUMMCR [49] . Briefly, for Kras allele, the imported mESC was HEPD0073_1_E09 (JM8.F6 ES cells). This cell line carries Kras tm1a(EUCOMM)Hmgu , a knockout of the first allele of the Kras gene (Ensembl ID: ENSMUSG00000030265 in Genome Assembly GRCm39). This allele places loxP sites on either side of exon 3 (ENSMUSE00000545805) of the mouse Kras gene transcript (Ensembl Transcript ID: Kras-201; ENSMUST00000032399.12). The presence of the isolated 3′ loxP site was confirmed by PCR using 5′-GTT ACA GCA GTT ACA TGA CTT GTC C-3′ and 5′-TTA AGG TCA TTG GAG TAA CAC CAT C-3′ (212bp). Following confirmation of correctly targeted clone for the Kras allele, mouse lines were derived by injection of targeted mESCs cells into Balb/c blastocysts according to standard protocols [50] . Chimeras were identified by black coat colour. For Braf , the mESC imported was EPD0608_5_D04 (JM8A3.N1 ES cells). This cell line carries Braf tm1a(EUCOMM)Wtsi , a knockout of the first allele of the Braf gene (Ensembl ID: ENSMUSG00000002413 in Genome Assembly GRCm39). The allele places loxP sites on either side of exon 5 (ENSMUSE00000618030) of Braf gene transcript (Ensembl Transcript ID: Braf -201; ENSMUST00000002487.15). The presence of the isolated 3′ loxP site was confirmed by PCR using 5′- GTT CGA GAC AGT CTA AAG AAA GCA C-3′ and 5′- GGC ATT TGT CAT AGG AAT AAA CAA C-3′ (513bp). Following confirmation of correctly targeted clone for the Braf allele, mouse lines were derived by injection of targeted mESCs cells into C57BL/6J blastocysts according to standard protocols [50] . Chimeras were identified by agouti coat colour. After breeding of the Kras and Braf chimeras, germline offspring were identified by coat colour and the presence of the modified allele was confirmed with the allele-specific 3′ loxP primers described above. To generate conditional alleles (tm1c) from the original knockout first allele (tm1a), both strains were subsequently crossed with a mouse strain expressing FLPe (Tg(ACTFLPe)9205Dym) to delete the selectable markers by recombination at the FRT sites [49] . Correct deletion of the selectable marker was confirmed by PCR across the remaining FRT site, using the oligos for Kras: 5′- ATT CAC AGT GTT GTG TGA CCA TTA G-3’ and 5′- AGT GAG ACC TTG TCT TAA TGC ACT C-3′ (432bp); and for Braf 5′- ACA CTC AGC TTT TTA GTG GGT ACT G-3′ and 5′- TTC CAC CAC TGA AAA TAC TTA AAG G-3′ (486bp). Following successful validation of the mouse strains carrying the Kras and Braf conditional alleles, genotyping was subsequently carried out by a commercial genotyping service provider (Transnetyx). Immunohistochemistry (IHC) and RNAscope Haematoxylin-and-eosin (H&E) staining was performed using standard protocols. Immunohistochemistry - IHC for BrdU (1:200, BD Biosciences #347580), β-catenin (1:50, BD Biosciences #610154), γ-H2AX (1:50, Cell Signalling Technologies #9718), phospho-ERK1/2 (1:400, Cell Signalling Technologies #9101), c-MYC (1:200 Abcam #ab32072), Lysozyme (1:300, Dako/Agilent #A099), αSMA (1:25000, Sigma-Aldrich #A2547), CD3 (1:100, Abcam #ab16669), CD4 (1:500, eBisoscience #14-9766-82), CD8 (1:500, eBisoscience #14-0808-82), F4/80 (1:200, Abcam #ab6640) and S100A9 (1:1500, CST #73425) was performed on formalin-fixed intestinal sections using standard protocols. Secondary antibodies used were EnVision anti-rabbit (undiluted, DAKO #K4003) and anti-mouse (undiluted, DAKO #K4001). All antibodies were commercially sourced, and validated by the manufacturer. In situ hybridisation (ISH) (RNAscope) was performed according to the manufacturer’s protocol (Advanced Cell Diagnostics RNAscope 2.0 High Definition–Brown) for Notum, Cxcl5 and Tgfb2 . Sections were counterstained with hematoxylin and coverslipped using DPX mountant (CellPath, UK). Picrosirius Red staining technique was used to stain collagen within tissue sections [32] . Assaying proliferation in vivo Proliferation levels were assessed by measuring BrdU incorporation. Mice were injected with 250 µl of BrdU (Amersham Biosciences) 2 h before being sacrificed. IHC staining for BrdU was then performed using an anti-BrdU antibody. For each analysis, 25 half-crypts were scored from at least three mice of each genotype. Cell lines and crypt culture Intestinal organoids were generated in-house from genetically engineered mouse models described above, with genotyping information provided by Transnetyx (Cordoba, TN, USA). Briefly, small intestinal and colon lines were generated from mice 3 days post tamoxifen induction. Small intestine and colon were scraped with a glass cover slip and washed repeatedly with cold PBS. Following 30 min EDTA incubation at 4 °C, crypts were isolated from tissue through mechanical pipetting, strained and cell pellets subsequently cultured in Matrigel and Advanced Dulbecco’s Modified Eagle Medium/Ham’s F-12 (Advanced DMEM/F-12, Gibco #12634010) supplemented with 2 mM L-glutamine (Gibco #A2916801), HEPES (Gibco #15630080) and 1% Penicillin-Streptomycin (Gibco #15070063). For tumour culture, a central piece of intestinal tumour was removed on dissection, washed in cold PBS and fragmented. Fragments were incubated in DNase and trypsin for 30 min and thoroughly dissociated. Advanced DMEM/F-12 media was added and the suspension pelleted. Following resuspension and straining cell pellets were cultured in Matrigel as above. ddPCR Genomic DNA was extracted from snap-frozen cell pellets or mouse tissues using the QIAGEN DNeasy Blood and Tissue Kit. Reactions were performed with ddPCRSupermix and primers and probes (Bio-Rad) listed below. ddPCR was carried out according to Bio-Rad’s protocol. Droplets were generated on Bio-Rad’s QX200 with droplet generation oil, subjected to amplification (95 °C 10 min, 94 °C 30 s, 59 °C 1 min, repeated 40×, 98 °C 10 minutes, 8 °C hold), and read on Bio-Rad’s QX200 Droplet Reader running QuantaSoft software. Primer sequences are as follows: KRAS_G12D Forward: CTGCTGAAAATGA-CTGAGTA, Reverse: ATTAGCTGTATCGTCAAGG, Probe:TGGAGCTGATGGCGT with FAM fluorophore; KRAS_wt Forward: CTGCTGAAAATGA-CTGAGTA, Reverse: ATTA GCTGTATCGTCAAGG, Probe Sequence: TGGAGCTGGT-GGCG with HEX fluorophore. RAS-activation assay Organoids were plated two days prior to the assay in Matrigel. For starvation, organoids were washed with PBS and fed ADF without EGF was for 30 min. After starvation organoids were quickly washed with ice-cold PBS, collected and disrupted prior to cell lysis. The following steps were performed using the Cytoskeleton RAS-activation assay biochem kit (#BK008) according to the manufacturer’s instructions. RNA extraction, qRT-PCR and RNA-sequencing RNA was extracted from whole tissue, organoids or tumour tissues using QIAGEN RNAeasy kit (Cat no. 74104) according to the manufacturer’s instructions. 1 µg of total RNA was reverse transcribed to cDNA using a High-Capacity cDNA Reverse Transcription Kit (Thermo Scientific, Cat 4368814). qPCR was performed in duplicates for each biological replicate in a 20 µl reaction, with 10 µl of 2X DyNAmoHSmaster mix (Thermo Scientific, Cat no. F410L), 2 µl cDNA and 0.5mM of each of the primers. The reaction mixture without a template was run in duplicate as a control. Gapdh was used to normalise for differences in RNA input. For RNA sequencing, RNA integrity was analysed using NanoChip (Agilent RNA 6000 Nano kit, 5067-1511). A total of 2 µg RNA was purified by poly(A) selection. The libraries were run on the Illumina NextSeq 500 using the High Output (75 cycles) kit (2 × 36 cycles, paired-end reads, single index). Analysis of RNA-seq data was carried out as previously described [51] . Geneset enrichment analysis was performed using GSEA version 4.1.0 software (Broad Institute). SDS-PAGE and western blotting Organoid pellets were washed in ice-cold PBS and lysed in RIPA buffer. Protein concentration was determined using BCA protein assay (Thermo scientific # 23225). 20ug protein were separated on a 4–12% gradient pre-cast gel (Novex #NP0322PK2) in MOPS running buffer. Samples were transferred onto PVDF membrane (Millipore, #IPFL00010). Primary antibodies were diluted as indicated in 5% BSA/TBS-T (Sigma #A9647) and incubated overnight at 4 °C (KRASG12D 1:1000, CST #14429; ß-actin 1:2000, SIGMA #A2228, ERK1/2 1:1000, CST #4695; pERK1/2 1:1000, CST #9101, MEK1/2 1:1000, CST ##8727 pMEK1/2 1:1000, CST #2338; AKT 1:1000, CST #9272; pAKT (Ser473) 1:2000, CST #4060, PTEN 1:1000, CST #9559). Secondary antibody (goat α-rabbit HRP, Dako #P0448, goat α-mouse HRP Dako #P0447) was diluted 1:2000 in 5% BSA/TBS-T and incubated for 1h at RT. All antibodies were commercially sourced, and validated by the manufacturer. Statistics Statistical analyses were performed using GraphPad Prism (v8) software (La Jolla, CA, USA). Statistical comparisons for survival data were performed using Mantel-Cox (Log-Rank) test. Mann–Whitney- U tests were performed using GraphPad Prism. In each figure legend, the data and errors are shown, and the relevant statistical test is specified. Reporting summary Further information on research design is available in the Nature Portfolio Reporting Summary linked to this article.